Sleep disruption impairs haematopoietic stem cell transplantation in mice Many of the factors affecting the success of haematopoietic cell transplantation are still unknown. Here we show in mice that donor sleep deprivation reduces the ability of its haematopoietic stem cells (HSCs) to engraft and reconstitute the blood and bone marrow of an irradiated recipient by more than 50%. We demonstrate that sleep deprivation downregulates the expression of microRNA (miR)-19b, a negative regulator of the suppressor of cytokine signalling (SOCS) genes, which inhibit HSC migration and homing. Accordingly, HSCs from sleep-deprived mice have higher levels of SOCS genes expression, lower migration capacity in vitro and reduced homing to the bone marrow in vivo . Recovery of sleep after sleep deprivation restored the reconstitution potential of the HSCs. Taken together, this study provides insights into cellular and molecular mechanisms underlying the effects of sleep deprivation on HSCs, emphasizing the potentially critical role of donor sleep in the success of bone marrow transplantation. While haematopoietic cell transplantation is a standard therapeutic procedure for various malignant and non-malignant diseases, the impact of sleep on haematopoietic cell transplantation has not been investigated. Sleep disorders affect metabolism, endocrine system and immune response [1] , [2] , [3] , [4] . We hypothesized that also haematopoietic stem cells (HSCs) are affected by sleep deprivation. These cells are used in haematopoietic cell transplantation procedures and are responsible for the lifelong production and maintenance of all blood and immune cells. Our hypothesis is supported by increasing evidence of a circadian regulation of HSCs and of the haematopoietic niche [5] , [6] , [7] . Circadian rhythms provide temporal organization to molecular, cellular and biochemical processes, and they may therefore be synchronizing HSC functions with sleep. A relationship of this nature between sleep and the function of HSCs can be especially important, as more than 100 million people around the world, including potential bone marrow (BM) donors, suffer from disorders of sleep and wakefulness. Nevertheless, no studies, thus far, have linked donor sleep profile with haematopoietic cell transplantation outcomes. This work focuses on the effects of sleep deprivation on the functions of HSCs. We show that 4 h of sleep deprivation in mice reduces the ability of HSCs to engraft and reconstitute the blood and BM of an irradiated recipient by more than 50%. We attribute these effects to an attenuated responsiveness of the HSCs to migration-guiding cues ex vivo and in vivo . At the cellular level, we show that sleep deprivation downregulates the expression of microRNA (miR)-19b, which is a negative regulator of the suppressor of cytokine signalling (SOCS) genes that inhibit HSC migration and homing. Using a standard luciferase reporter assay, we validate in vitro the interaction between miR-19b and SOCS3 and demonstrate that sleep deprivation elevates SOCS3 levels. Using genetic manipulations, we demonstrate that in the absence of SOCS3 sleep deprivation does not significantly affect HSC migration. Finally, we show that growth hormone (GH) levels, which are regulated by sleep, alter miR-19b concentrations in HSCs and affect HSC migration. Thus, representing a possible mechanism mediating the effects of sleep deprivation on HSCs. Reduction in reconstitution potential following sleep deprivation To determine the effects of sleep deprivation on HSC transplantation potential, mice were allowed to sleep ad libitum for 4 h (Zeitgeber time (ZT) ZT0–ZT4; sleep) or were sleep-deprived for the same duration by gentle handling. The efficiency of the sleep deprivation protocol was monitored by electroencephalography (EEG) and electromyography (EMG; Fig. 1a ). Gentle handling was chosen as the means of depriving mice of sleep, so as to avoid stress [8] . In line with previous studies [8] , there was no difference in plasma corticosterone (Cort) levels between the two experimental groups ( Fig. 1b ; Student’s t -test; P =0.6814; df=10; t =0.422). All animals were examined at the same circadian time to rule out a potential direct circadian contribution to the observed effects. 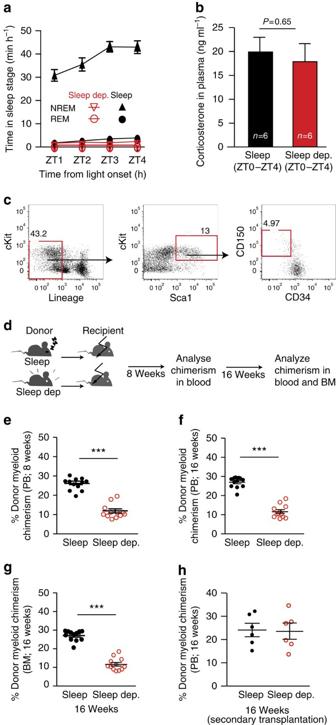Figure 1: HSCs isolated from sleep-deprived mice have reduced mid-term and long-term reconstitution potential in lethally irradiated hosts. (a) Mice were sleep-deprived, by gentle handling, for 4 h, immediately after light onset (ZT0–ZT4;n=8 per group). REM and non-REM duration were determined using EEG and EMG, individually plotted for each hour (sleep-deprived points in red; mean±s.e.m). (b) Plasma of the sleep and sleep-deprived mice was analysed using ELISA for corticosterone levels (n=8 per group; mean±s.e.m). (c) We isolated HSCs from mice that were allowed to sleep or from sleep-deprived mice. The flow cytometry gating scheme for HSC isolation is shown on a representative mouse. (d) To test the mid-term and long-term transplantation potential of the isolated HSCs, we intravenously injected 300 HSC mice into lethally irradiated congenic recipients (to distinguish between the donor and recipient cells, we used CD45.1 mice as donors and CD45.2 as recipients). Peripheral blood (PB) samples were collected from the recipient mice at (e) 8 weeks (PB), (f) 16 weeks and (g) BM post transplantation. Cells were analysed for myeloid chimerism, as determined by the percentage of myeloid cells derived from the donor compared with the total number of myeloid cells in the indicated tissue (mean±s.e.m; Student’st-test; ***P<0.0001). In all experiments, HSCs were transplanted along with 1 × 106bone marrow mononuclear cells to support mouse survival ((d–g)n=12 mice per group). (h) Primary recipients received HSCs from sleep or sleep-deprived donors as indicated ind–g. Then, at 16 weeks, 2.5 × 106BM cells from primary recipients were transplanted into a new group of lethally irradiated CD45.2+ (secondary recipients), and donor-derived reconstitution was assessed in the secondary recipients (mean±s.e.m; Student’st-test;P=0.83) Figure 1: HSCs isolated from sleep-deprived mice have reduced mid-term and long-term reconstitution potential in lethally irradiated hosts. ( a ) Mice were sleep-deprived, by gentle handling, for 4 h, immediately after light onset (ZT0–ZT4; n =8 per group). REM and non-REM duration were determined using EEG and EMG, individually plotted for each hour (sleep-deprived points in red; mean±s.e.m). ( b ) Plasma of the sleep and sleep-deprived mice was analysed using ELISA for corticosterone levels ( n =8 per group; mean±s.e.m). ( c ) We isolated HSCs from mice that were allowed to sleep or from sleep-deprived mice. The flow cytometry gating scheme for HSC isolation is shown on a representative mouse. ( d ) To test the mid-term and long-term transplantation potential of the isolated HSCs, we intravenously injected 300 HSC mice into lethally irradiated congenic recipients (to distinguish between the donor and recipient cells, we used CD45.1 mice as donors and CD45.2 as recipients). Peripheral blood (PB) samples were collected from the recipient mice at ( e ) 8 weeks (PB), ( f ) 16 weeks and ( g ) BM post transplantation. Cells were analysed for myeloid chimerism, as determined by the percentage of myeloid cells derived from the donor compared with the total number of myeloid cells in the indicated tissue (mean±s.e.m; Student’s t -test; *** P <0.0001). In all experiments, HSCs were transplanted along with 1 × 10 6 bone marrow mononuclear cells to support mouse survival (( d – g ) n =12 mice per group). ( h ) Primary recipients received HSCs from sleep or sleep-deprived donors as indicated in d – g . Then, at 16 weeks, 2.5 × 10 6 BM cells from primary recipients were transplanted into a new group of lethally irradiated CD45.2+ (secondary recipients), and donor-derived reconstitution was assessed in the secondary recipients (mean±s.e.m; Student’s t -test; P =0.83) Full size image To test the transplantation potential of HSCs derived from mice that were allowed to sleep and sleep-deprived mice, 300 HSCs (lin−, c-kit+, Sca-1+, CD34−, CD150+; Fig. 1c ) were isolated by fluorescence-activated cell sorting (FACS) from the BM of the two groups and intravenously transplanted into lethally irradiated recipient mice, along with 1 × 10 6 BM-derived mononuclear cells to support recipient survival. Support cells were isolated from CD45.2+ mice (the recipients) that were allowed to sleep normally (the same pool of cells was used for both experimental groups). Reconstitution potential of transplanted HSCs was measured 8 and 16 weeks thereafter. The percentage of donor myeloid cells in the peripheral blood of the recipient was assessed, as a proxy for HSC chimerism [9] . Transplantation efficiency at 8 and 16 weeks was lower for HSCs derived from sleep-deprived mice ( Fig. 1d–g ). At 16 weeks post transplantation, donor myeloid chimerism was 26.42±0.8% in mice that received HSCs from mice that were allowed to sleep compared with 11.62±1% in mice that received HSCs from sleep-deprived mice (Student’s t -test; t (22)=10.77; P <0.0001). Because all recipient mice underwent the same treatment before transplantation, we concluded that these effects were intrinsic to donor HSCs. To discern between short-term and long-term effects of sleep deprivation on the reconstitution potential of HSCs, we performed secondary transplantation experiments ( Fig. 1h ). In these experiments, the chimeric mice that received the initial BM transplantation from either mice that were allowed to sleep or sleep-deprived mice served as the donors for the secondary transplantation. These secondary donors were not subjected to any sleep manipulation. Analysis of the donor myeloid chimerism in the secondary transplantation recipients did not identify any difference between the two groups. This suggested that sleep deprivation induced a temporary change in the reconstitution potential of HSCs, which recovered by 16 weeks post transplantation. HSCs from sleep-deprived mice have reduced homing capacity Reconstitution of the haematopoietic system following transplantation requires homing of HSCs from the peripheral blood to their supported niche in the BM [10] , [11] . To determine whether the homing potential of HSCs was affected by sleep deprivation, donor HSCs were traced in vivo after transplantation. HSCs were isolated from the BM of green fluorescence protein (GFP)-expressing transgenic mice that were either allowed to sleep ad libitum or were sleep-deprived for 4 h. The GFP-expressing HSCs were then intravenously administered to lethally irradiated congenic, non-GFP-expressing recipient mice. Twelve hours later, the mice were killed and the number of GFP-expressing cells that successfully homed and localized to the BM was determined. Fewer HSCs from sleep-deprived mice homed to the BM during this time period, when compared with HSCs from control mice ( Fig. 2a,b ; 3.3±1.4% mice allowed to sleep; 1.7±0.3% sleep-deprived mice; Student’s t -test; P <0.05). These findings show that HSCs from sleep-deprived mice are indeed impaired in their homing potential, a crucial component in the success of haematopoietic cell transplantation [10] , [11] . 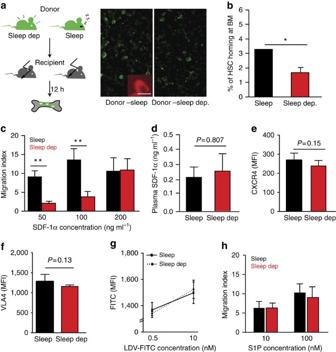Figure 2: HSCs from sleep-deprived mice have reduced homing capacityin vivoandin vitro. (a) HSCs derived from GFP-expressing, sleep-deprived mice were transplanted into lethally irradiated congenic mice that did not express GFP (control mice were allowed to sleep for the same duration). The donor HSCs were visualized 12 h later in the recipient’s bone under a fluorescence microscope. GFP expression was validated using anti-GFP staining and a representative image is shown in the insert. Scale bar, 10 μm (n=6–11 mice per group; mean±s.e.m.). (b) The number of GFP-labelled cells in the recipient’s BM was determined. Results are presented as the percentage of homing, assuming that two tibias and two femurs represent 20% of total mouse BM (Student’st-test; P=0.021;t=2.56; df=15). (c) Migration towards SDF-1α was determinedin vitrousing a transwell migration assay. KLS cells were placed in the upper chamber and the chemoattractant (SDF-1α, 50, 100 or 200 ng ml−1) was immersed in the medium of the lower chamber. Migration across the membrane in response to the chemoattractant was determined using flow cytometry, after 4 h of incubation, and compared with baseline migration in the absence of the chemoattractant. Results are presented as a migration index (50 ng ml−1SDF-1α: 9.6±1.7% in the sleep group compared with 2.06±0.4% in the sleep-deprived group; 100 ng ml−1SDF-1α: 14.5±3.4% in the sleep compared with 3.6±1.4% in the sleep-deprived mice; repeated measures ANOVA sleep:F(2,15)=10.18,P<0.0061;n=6 mice per group; mean±s.e.m. (d) Plasma was collected and analysed using ELISA for SDF-1α levels, from sleep or sleep-deprived mice. (e) CXCR4 levels on HSCs derived from sleep and sleep-deprived mice (mean fluorescent intensity (MFI)±s.e.m). (f) VLA4 (α4) levels on HSCs derived from sleep and sleep-deprived mice. (g) Cells were cultured with 0.5 or 10 nM LDV-FITC to evaluate VLA4-binding affinity. Binding was evaluated as FITC MFI on HSCs (mean±s.e.m). Statistical significance was determined by Student’st-test. (h) Migration towards S1P was determinedin vitrousing a transwell migration assay as described inc. S1P concentration is indicated. Repeated measure ANOVA (n=4 mice per group) (*P<0.05; **P<0.001). Figure 2: HSCs from sleep-deprived mice have reduced homing capacity in vivo and in vitro . ( a ) HSCs derived from GFP-expressing, sleep-deprived mice were transplanted into lethally irradiated congenic mice that did not express GFP (control mice were allowed to sleep for the same duration). The donor HSCs were visualized 12 h later in the recipient’s bone under a fluorescence microscope. GFP expression was validated using anti-GFP staining and a representative image is shown in the insert. Scale bar, 10 μm ( n =6–11 mice per group; mean±s.e.m.). ( b ) The number of GFP-labelled cells in the recipient’s BM was determined. Results are presented as the percentage of homing, assuming that two tibias and two femurs represent 20% of total mouse BM (Student’s t -test ; P =0.021; t =2.56; df=15). ( c ) Migration towards SDF-1α was determined in vitro using a transwell migration assay. KLS cells were placed in the upper chamber and the chemoattractant (SDF-1α, 50, 100 or 200 ng ml −1 ) was immersed in the medium of the lower chamber. Migration across the membrane in response to the chemoattractant was determined using flow cytometry, after 4 h of incubation, and compared with baseline migration in the absence of the chemoattractant. Results are presented as a migration index (50 ng ml −1 SDF-1α: 9.6±1.7% in the sleep group compared with 2.06±0.4% in the sleep-deprived group; 100 ng ml −1 SDF-1α: 14.5±3.4% in the sleep compared with 3.6±1.4% in the sleep-deprived mice; repeated measures ANOVA sleep: F (2,15)=10.18, P <0.0061; n =6 mice per group; mean±s.e.m. ( d ) Plasma was collected and analysed using ELISA for SDF-1α levels, from sleep or sleep-deprived mice. ( e ) CXCR4 levels on HSCs derived from sleep and sleep-deprived mice (mean fluorescent intensity (MFI)±s.e.m). ( f ) VLA4 (α4) levels on HSCs derived from sleep and sleep-deprived mice. ( g ) Cells were cultured with 0.5 or 10 nM LDV-FITC to evaluate VLA4-binding affinity. Binding was evaluated as FITC MFI on HSCs (mean±s.e.m). Statistical significance was determined by Student’s t -test. ( h ) Migration towards S1P was determined in vitro using a transwell migration assay as described in c . S1P concentration is indicated. Repeated measure ANOVA ( n =4 mice per group) (* P <0.05; ** P <0.001). Full size image Migration of the HSCs towards guiding cues is required for their effective homing to the BM. To determine whether the migration capacity of the HSCs is affected by sleep, we performed a transwell migration assay ( Fig. 2c ) and compared the number of HSCs migrating towards different concentrations of the migration-guiding chemokine, stromal cell-derived factor-α (SDF-1α). Migration towards low concentrations of SDF-1α (50–100 ng ml −1 ) was significantly decreased in HSCs derived from sleep-deprived mice, compared with HSCs derived from mice that were allowed to sleep. Interestingly, no differences in HSC migratory potential to a higher SDF-1α concentration (200 ng ml −1 ) were observed. This suggested that the HSCs of sleep-deprived mice do not lose their inherent ability to migrate towards SDF-1α, but rather require a higher threshold of SDF-1α for migration. We could not explain this effect by changes in SDF-1α levels ( Fig. 2d ) or in the levels of CXCR4, the cell-surface receptor for SDF-1α (ref. 12 ), which were comparable between the experimental groups ( Fig. 2e ). There was also no difference between the mice that were allowed to sleep and sleep-deprived mice in the levels of Very Late Antigen-4 (VLA4) integrin (alpha4 unit; Fig. 2f ) or its binding affinity ( Fig. 2g ). Moreover, migration towards sphingosine-1-phosphate (S1P), a chemotactic agent present in the blood and known to support HSCs egress from the BM to the blood, was also unaffected by sleep deprivation ( Fig. 2h ). These findings indicate that the overall motility potential of the cells was not affected by sleep deprivation, suggesting that the impaired localization of the HSCs to the BM was mediated by specific change in the responsiveness to migration-guiding cues, especially SDF-1α. Sleep deprivation alters miR-19b and SOCS3 mRNA levels Post-transcriptional changes within the HSCs derived from mice that were allowed to sleep or following sleep deprivation were analysed in efforts to identify intracellular changes occurring in the HSCs. We were looking for changes that could explain the altered HSC in vitro migration to SDF-1α, in vivo homing following transplantation and the overall reduced transplantation potential. miRs are noncoding RNA molecules that repress transcriptional outputs in a sequence-dependent manner [13] . It was previously shown that sleep loss alters miR expression in the brain [14] . We profiled the expression of a panel of 376 highly conserved and well-known miRs. Data were normalized to U6 expression, which had similar C t values. Values for other controls, snoRNA-202 and snoRNA-135, were also comparable; therefore, differences in miR expression were not attributable to changes in controls. Of the 376 miRs in the array, 98 miRs were amplified ( C t <35). Comparative analysis of expression levels between HSCs derived from sleep-deprived mice or mice that were allowed to sleep revealed an overall downregulation of miRs ( Fig. 3a ; public deposit at GEO; GSE48144), where 67% of the normally amplified miRs were downregulated in HSCs from sleep-deprived mice, while 8% were further amplified in HSCs derived from sleep-deprived mice. Comparable levels were observed between the two groups for 24% of the tested miRs. Single TaqMan probes were used for specific miRs to validate the array ( Supplementary Fig. 1 ). In the downregulated set of miRs, miR-152 and miR-361 were downregulated by eightfold in cells from sleep-deprived mice. However, these miRs were amplified with high C t values, suggesting that they were not abundant in HSCs and we therefore did not focus on these miRs. Nevertheless, several members of the miR-17 family were downregulated. The miR-17 family includes miR-17, miR-18a, miR-19a, miR-20a, 19b-1 and miR-92a-1, which are transcribed from the same polycistron and in the same genomic context (in mice it is chromosome 14). In both samples, miR-17, miR-19b and miR-92 were the most abundant miRs in the cluster ( C t <25), and miR-18a/b were the least abundant ( C t >35). miR-19b displayed the greatest fold change (fourfold decrease) in the cluster on sleep deprivation and we therefore focused on that miR. 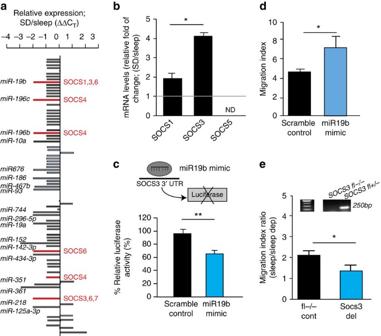Figure 3: Sleep deprivation decreases the levels of miR-19b and increases the levels of SOSC3 in HSCs. (a) miR profiles of HSCs from sleep and sleep-deprived mice were analysed by multiplex quantitative real-time PCR after HSC sorting by FACS. The ΔΔCtmethod was used, with U6, sno-202 and sno-135 as normal controls. miR levels underwent more than fourfold changes and potentially targeted SOCS genes are highlighted. (b) qPCR analysis of SOCS1, SOCS3 and SOCS5 levels. Results are presented as fold change normalized to GAPDH (ND=not detected; three independent repeats,n=4 mice per group; SOCS3: 4.13±0.5-fold and SOCS1: 1.9±0.8-fold). (c) A schematic presentation of the luciferase reporter system in 293T cells that were transfected with a miR mimic or scramble control and pMir Target construct containing the 3′UTR of SOCS3 and an RFP reporter. Luciferase activity was measured 48 h after transfection and normalized to RFP and then to the values measured for vector alone (Student’st-test;t(4)=8.313;P=0.0011; mean±s.e.m.). (d) Migration of HSCs, transfected with 50 nM miR-19b mimic or scramble control, towards 50 ng ml−1SDF-1α. Migration was compared with baseline migration in the absence of chemoattractant (migration index). (e) Mx-1 cre mice were crossed with SOCS3-floxed mice. Mx-1 cre mice express Cre recombinase under the control of an inducible Mx-1 promoter, active after induction with polyinosinic–polycytidylic acid (pI:pC). When bred with SOCS3-floxed mice (carrying SOCS3 gene flanked by loxP recognition sites), the expression of Cre recombinase causes SOCS3 gene deletion. Upper panel: genomic DNA was extracted from FACS-sorted KLS cells and analysed using PCR. The PCR product obtained from the SOCS fl+ locus is 250-bp band indicates cre-mediated deletion of SOCS3 (SOCS3del). Lower panel: migration of KLS cells isolated from sleep mice and from mice that were deprived of sleep for 4 h. We compared two sets of mice, mice that express mx-1 cre and SOCS3- floxed gene and their littermates that do not express mx-1 cre. This allows controlling for potential effect of pI:pC injection required to induce cre expression. Migration towards 50 ng ml−1SDF-1 α was determined for cells from sleep or sleep-deprived mice. The migration index was determined for each group, and the ratio between the migration index of the control and the SOCS-3-deleted mice was calculated (mean±s.e.m). Sleep deprivation (SD); (*P<0.05; **P<0.01). Figure 3: Sleep deprivation decreases the levels of miR-19b and increases the levels of SOSC3 in HSCs. ( a ) miR profiles of HSCs from sleep and sleep-deprived mice were analysed by multiplex quantitative real-time PCR after HSC sorting by FACS. The ΔΔ C t method was used, with U6, sno-202 and sno-135 as normal controls. miR levels underwent more than fourfold changes and potentially targeted SOCS genes are highlighted. ( b ) qPCR analysis of SOCS1, SOCS3 and SOCS5 levels. Results are presented as fold change normalized to GAPDH (ND=not detected; three independent repeats, n =4 mice per group; SOCS3: 4.13±0.5-fold and SOCS1: 1.9±0.8-fold). ( c ) A schematic presentation of the luciferase reporter system in 293T cells that were transfected with a miR mimic or scramble control and pMir Target construct containing the 3′UTR of SOCS3 and an RFP reporter. Luciferase activity was measured 48 h after transfection and normalized to RFP and then to the values measured for vector alone (Student’s t -test; t (4)=8.313; P =0.0011; mean±s.e.m.). ( d ) Migration of HSCs, transfected with 50 nM miR-19b mimic or scramble control, towards 50 ng ml −1 SDF-1α. Migration was compared with baseline migration in the absence of chemoattractant (migration index). ( e ) Mx-1 cre mice were crossed with SOCS3-floxed mice. Mx-1 cre mice express Cre recombinase under the control of an inducible Mx-1 promoter, active after induction with polyinosinic–polycytidylic acid (pI:pC). When bred with SOCS3-floxed mice (carrying SOCS3 gene flanked by loxP recognition sites), the expression of Cre recombinase causes SOCS3 gene deletion. Upper panel: genomic DNA was extracted from FACS-sorted KLS cells and analysed using PCR. The PCR product obtained from the SOCS fl+ locus is 250-bp band indicates cre-mediated deletion of SOCS3 (SOCS3del). Lower panel: migration of KLS cells isolated from sleep mice and from mice that were deprived of sleep for 4 h. We compared two sets of mice, mice that express mx-1 cre and SOCS3- floxed gene and their littermates that do not express mx-1 cre. This allows controlling for potential effect of pI:pC injection required to induce cre expression. Migration towards 50 ng ml −1 SDF-1 α was determined for cells from sleep or sleep-deprived mice. The migration index was determined for each group, and the ratio between the migration index of the control and the SOCS-3-deleted mice was calculated (mean±s.e.m). Sleep deprivation (SD); (* P <0.05; ** P <0.01). Full size image The highly conserved SOCS3, a protein previously implicated in HSC migration [15] , [16] , [17] , was predicted using Targetscan to be a miR-19b target. Thus, we compared the levels of SOCS gene expression in our experimental groups reasoning that decreases in miR levels can result in the stabilization of otherwise degraded transcripts. A twofold increase in SOCS1 and a fourfold increase in SOCS3 mRNA levels were observed in HSCs from sleep-deprived mice, relative to HSCs from mice that were allowed to sleep ( Fig. 3b ). We did not detect a significant difference in mRNA levels of another miR-19b target, Pten, and we therefore focused on SOCS genes and specifically analysed the interaction of miR-19b with SOCS3. To validate the interaction between miR-19b and SOCS3, we performed a standard luciferase reporter assay. We used 293T cells transfected with a reporter containing the 3′-untranslated repeat (UTR) of SOCS3 ( Fig. 3c ). In this test, if the manipulated miR (miR-19b) binds the 3′UTR of the target gene (SOCS3) it reduces luciferase activity. A significant reduction in luciferase activity was measured among 293T cells transfected with a miR-19b mimic for 48 h, demonstrating that miR-19b interacts with the 3′UTR of SOCS3. Taken together, these findings indicate that sleep deprivation decreases miR-19b levels and upregulates SOCS3 gene expression levels in HSCs. To establish a functional connection between these changes in miR-19b and altered HSC migration capacity, we transfected KLS (c-kit+, Lin−, Sca+) cells from naive mice with miR-19b mimic for 36 h and tested their migration capacity towards SDF-1α. We used KLS cells because of the technical limitation of performing such manipulation on HSCs. In line with evidence obtained in other cell types [18] , miR-19b mimic increased HSC migration towards SDF-1α ( Fig. 3d ; Student’s t -test P =0.0195). This evidence indicates that the change in miR-19b levels can explain at least partially the reduced migration capacity of HSCs following sleep deprivation. The involvement of SOCS3 in HSC migration has been manifested before [15] , [16] , [17] . Yet, to directly test whether the effects of sleep deprivation on SOCS3 levels could affect the motility of these cells, we used a Cre recombinase under the control of the Mx-1 promoter to induce the deletion of SOCS3 gene in multiple cell types including BM cells. We found that HSCs from mice that had reduced levels of SOCS3 expression did not demonstrate a significant sleep-deprivation-associated impairment of migratory capacity when compared with controls ( Fig. 3e ; Student’s t -test P =0.017). Although there are some limitations to this experimental paradigm, these findings suggest that the effect of sleep deprivation on HSC migration is mediated at least in part via SOCS3. GH affects miR-19b expression and cell migration The effects of sleep deprivation on the HSCs raise questions regarding the identity of the signal from the sleeping brain to the haematopoietic system. One potential candidate is GH, which is secreted during sleep. GH has been shown to regulate lymphocyte migration [19] and increase mobilization of HSCs in humans [20] . GH receptors (GHR) are expressed in all murine haematopoietic tissues, especially in the BM [21] . In line with previous evidence [22] , we found that the sleep-dependent increase in GH levels was attenuated in sleep-deprived mice ( Fig. 4a ; one-way analysis of variance (ANOVA) F (2,22)=8.44; P =0.0019; Tukey post hoc comparisons P <0.01 for the light onset compared with the group of mice allowed to sleep; P <0.05 for mice allowed to sleep compared with sleep-deprived mice). To determine whether GH can mediate the observed changes in miR levels, HSCs were incubated with GH for 30 min and RNA was extracted immediately thereafter. We focused on the expression of miRs encoded by the miR-17 cluster, which includes miR-19b. The GH treatment led to an elevation in the levels of miR-19b and other members of the cluster, suggesting that GH may regulate the expression of this polycistron during sleep ( Fig. 4b ). Moreover, GH treatment had a direct, dose-dependent (bell-shaped response) effect on the migration capacity of HSCs ( Fig. 4c ). Low doses of GH increased migration, whereas high doses of GH had the opposite effect by reducing HSC migration. These findings show that GH levels, which are regulated by sleep, alter miR-19b concentrations in HSCs and affect HSC migration. This may thus represent a possible mechanism mediating the effects of sleep deprivation on HSCs. 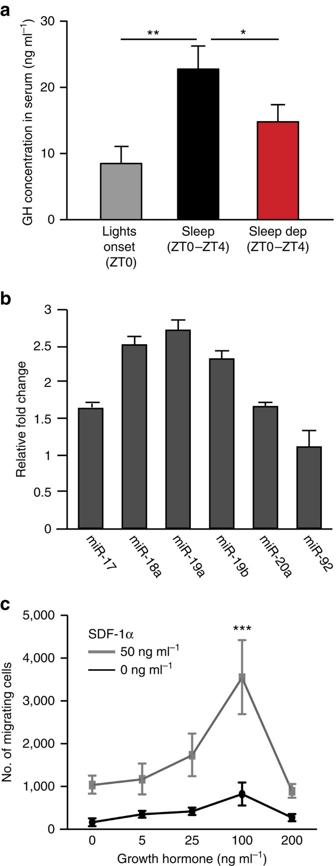Figure 4: Growth hormone alters the expression of miR-19b and cell migration. (a) Mice were either killed with light onset, after 1.5 h or 3 h of sleep deprivation or after 1.5 or 3 h of sleep, and plasma GH levels were determined using ELISA (one-way ANOVA followed by Tukey’s multiple comparisons test; mean±s.e.m). (b) KLS cells were treated with GH (100 ng ml−1dose was determined based on previous studies33,34) for 30 min, and RNA was extracted using Trizol for analysis of miR levels. All values were statistically significant within each group (technical replicas) and are reported as fold of change relative to control that was used as a reference (mean±s.e.m). (c) Cells from control mice were pre-incubated for 30 min with GH (0, 5, 25, 50 or 100 ng ml−1), washed and the migration of KLS to increasing concentrations of SDF-1α was determined on transwell migration plates. Statistical analyses were analysed using one-way ANOVA followed by Tukey’s multiple comparisons test; *P<0.05; **P<0.01; ***P<0.001;n=4 mice per group. Figure 4: Growth hormone alters the expression of miR-19b and cell migration. ( a ) Mice were either killed with light onset, after 1.5 h or 3 h of sleep deprivation or after 1.5 or 3 h of sleep, and plasma GH levels were determined using ELISA (one-way ANOVA followed by Tukey’s multiple comparisons test; mean±s.e.m). ( b ) KLS cells were treated with GH (100 ng ml −1 dose was determined based on previous studies [33] , [34] ) for 30 min, and RNA was extracted using Trizol for analysis of miR levels. All values were statistically significant within each group (technical replicas) and are reported as fold of change relative to control that was used as a reference (mean±s.e.m). ( c ) Cells from control mice were pre-incubated for 30 min with GH (0, 5, 25, 50 or 100 ng ml −1 ), washed and the migration of KLS to increasing concentrations of SDF-1α was determined on transwell migration plates. Statistical analyses were analysed using one-way ANOVA followed by Tukey’s multiple comparisons test; * P <0.05; ** P <0.01; *** P <0.001; n =4 mice per group. Full size image Sleep rebound restores the transplantation potential of HSCs Sleep is intensified after sleep deprivation and can often reverse processes impaired by sleep deprivation [23] . We tested whether recovery sleep can reverse the impaired transplantation potential of HSCs derived from sleep-deprived mice. Lethally irradiated congenic mice were transplanted with HSCs derived from (i) mice that were sleep-deprived for 4 h and allowed to recover their sleep for 2 h (ii) mice that were allowed to sleep for 6 h or (iii) mice that were sleep-deprived for 6 h. BM chimerism of recipient mice was analysed at 16 weeks post transplantation ( Fig. 5 ). Two hours of recovery sleep reversed the impaired transplantation capacity induced by sleep deprivation. Thus, HSCs from mice that were allowed to sleep and in the sleep-rebound group were equally potent in their transplantation potential. These findings suggest that controlling sleep can affect haematopoietic transplantation outcomes. 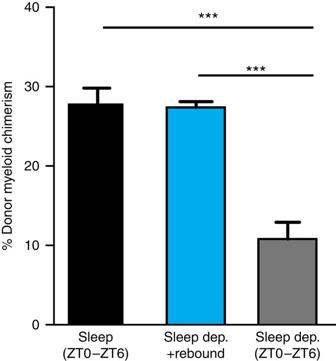Figure 5: Sleep rebound restores the reconstitution potential in lethally irradiated hosts. Chimerism in the BM of mice transplanted with HSC derived from mice that were allowed to recover their sleep for 2 h, mice deprived of sleep for 6 h and mice allowed to sleep for 6 h. Analysis of was performed at 16 weeks after transplantation (F(2,15)=192.9;P<0.0001). ***P<0.001. Mean±s.e.m.;n=6 mice per group. Figure 5: Sleep rebound restores the reconstitution potential in lethally irradiated hosts. Chimerism in the BM of mice transplanted with HSC derived from mice that were allowed to recover their sleep for 2 h, mice deprived of sleep for 6 h and mice allowed to sleep for 6 h. Analysis of was performed at 16 weeks after transplantation ( F (2,15)=192.9; P <0.0001). *** P <0.001. Mean±s.e.m. ; n =6 mice per group. Full size image This study demonstrates that sleep deprivation impairs the homing capacity and the reconstitution potential of transplanted HSCs. We show that this is a temporary effect, as secondary transplantation was not affected by the sleep deprivation. We attribute these effects of sleep deprivation on the transplantation potential to the reduced homing of the HSC to their niche in the BM as manifested in the in vivo homing assay. We further support the negative effects of sleep deprivation on HSC migration by demonstrating that the ex vivo migration capacity towards SDF-1α of the cells from sleep-deprived mice was reduced. We show that this was not due to changes in the receptor for SDF-1α, CXCR4 or changes in the levels of other integrins such as VLA4, but rather due to a change in the intracellular potential of the cells to respond to migration-guiding cues. We specifically show that cells derived from sleep-deprived mice have lower levels of miR-19b and increased SOCS3 levels, which was previously shown to affect migration to SDF-1α and stem cell trafficking [15] , [16] , [17] . We then used a genetic (Mx-1 Cre) manipulation to reduce SOCS3 levels in HSCs. We demonstrate that in the absence of SOCS3, sleep deprivation had no significant effect on the migration potential of HSCs, further supporting the role of SOCS3 in attenuating HSC migration following sleep deprivation. Finally, we show that sleep rebound reverses the effects of sleep deprivation on the transplantation potential of HSCs. Taken together, our findings indicate that even short-term sleep deprivation of a donor can affect the success of haematopoietic cell transplantation. These findings are especially relevant, as sleep deprivation is common even in healthy populations. Moreover, BM donors may experience acute sleep deprivation, partially due to the anticipation of the donation procedure, and partially due to the effect of pharmacological treatments. For example, it was shown that granulocyte colony-stimulating factor (G-CSF) suppresses sleep intensity manifested by reduced amount of slow-wave sleep and a reduction in the electroencephalographic delta power [24] . Yet, in this study we did not examine the effects of sleep deprivation on stem cell mobilization procedures. Nor did we analyse the potential effects of sleep deprivation on the routine circulation of HSCs between the BM and peripheral blood. As sleep is a complex phenomenon, it is difficult to determine the factors that mediate the effects of sleep on the reconstitution potential of the HSC. Sleep affects almost every physiological and behavioural system (metabolism, heart rate, endocrine system, immune system and so on [2] , [7] , [25] , [26] , [27] ). It is therefore unlikely that a single factor mediates all the effects of sleep on the haematopoietic system. Nevertheless, we propose GH as one possible mediator, particularly because its levels are regulated by sleep and, as we show, it can alter the levels of the miR-17 family, including miR-19b, in HSCs. These findings fall in line with previous studies indicating that GH regulates lymphocyte migration [19] as well as the mRNA expression and kinetics of suppressors of cytokine signalling (SOCS3) in several cell types [28] , [29] . Accordingly, GH is used to increase mobilization of HSCs in humans [20] and can be potentially applied to overcome the adverse effects of sleep deprivation on human haematopoietic cell transplantation efficacy. It is less likely that circadian mediators are responsible for the effects described in this study, as all experiments were performed at the same circadian phase and the sleep deprivation was for only 4 h. Moreover, CXCR4/SDF-1α levels, which have been previously implicated to mediate some of the circadian effects on HSCs [5] , [6] , [7] , were not affected in our experiments. We suggest that under normal conditions, both sleep and circadian factors affect HSC trafficking; circadian factors regulate SDF-1α levels [30] , while sleep controls intracellular SOCS levels. Long-term sleep deprivation (several days), or deprivation of specific sleep stages, has been shown to have additional, substantial effects on the haematopoietic system [4] . For example, a decrease in total cellularity of the BM and peripheral blood [4] , along with a decrease in the absolute number of haematopoietic stem/progenitor cells and colony-forming units, has been previously observed in mice that were deprived of rapid eye movement (REM) sleep for 72 h (ref. 4 ). The presented work demonstrated that sleep deprivation increases SOCS3 levels in HSCs. SOCS genes regulate the JAK/STAT pathway, which regulates the functions of various cytokines, including those used in mobilization and stimulation of the haematopoietic and immune systems, such as G-CSF, erythropoietin, thrombopoietin, interferons and numerous interleukins [31] . Sleep deprivation results in lower levels of miR-19b, stabilizing SOCS3 mRNA. Thus, we propose that a reduction in responsiveness to multiple cytokines, induced by an increase in SOCS levels, reduces HSC migration capacity and their homing from the blood to the BM after transplantation. It is also possible that sleep deprivation alters additional aspects of the HSC interaction with their BM niche (for example, the multilineage differentiation of the grafted cells). Thus, the specific molecular mechanism and the signals mediating the effects of sleep on the HSCs will require further detailed investigation. The current study provides evidence that sleep deprivation impairs haematopoietic cell transplantation potential. The potential implication of sleep deprivation of the donor may be crucial for the success of the fragile transplantation procedure. Our findings that sleep rebound can reverse the effects of sleep deprivation suggest that simple behavioural procedures can improve the success of BM transplantation. Animals All procedures were approved by the Stanford University Institutional Animal Care and Use Committee and were in compliance with the Guide for the Care and Use of Laboratory Animals. The donor mice were 8–12-week-old C57BL/6-CD45.1+ or GFP-transgenic C57BL/6-CD45.1+ mice. The recipient mice were 8–12-week-old C57BL/6-CD45.2 male mice. Animals were derived and maintained at the Stanford University’s Research Animal Facility or obtained from Jackson Laboratories. Environmental conditions were maintained at 24±1 °C, humidity 40–60% and light cycle 12/12 h. Food and water were provided ad libitum . Animals were killed using CO 2 . All groups were treated similarly to avoid potential difference in stress levels. Polysomnographic recording and data analysis Surgery . A custom-made EEG and EMG implant was surgically implanted under intraperitoneal ketamine/xylazine anaesthesia (80 and 16 mg kg −1 , respectively), using a small animal stereotaxic frame (David Kopf Instruments, CA, USA). EEG signals were recorded from electrodes placed over the frontal (anterior/posterior (AP), −2 mm; medial/lateral (ML), ±1 mm) and temporal (AP, 3 mm; ML, 2.5 mm) cortices. EMG signals were recorded from two electrodes inserted in the neck musculature. The implants were affixed to the skull with C&B Metabond (Parkell; Edgewood, NY) and dental acrylic. After the surgical procedure, animals were allowed to recover for at least 14 days. They were then acclimated to a flexible EEG/EMG connection cable for 7 days, within individual recording chambers and habituated daily to handling. Data acquisition EEG and EMG signals, detected by the surgically implanted electrodes, were collected using commercial hardware (Embla; Broomfield, CO), digitized at 256 Hz and visualized using a sleep-recording software Somnologica-3 (Medcare, Reykjavik, Iceland). Scoring Sleep was scored using the sleep analysis software (SleepSign for Animal; Kissei Comtec America). All scoring was performed manually on the basis of the visual signature of the EEG and EMG waveforms in 4-s epochs. Two independent investigators verified scoring criteria as follows: waking was defined as a predominance of fast, desynchronized waves and a high-EMG amplitude. Non-REM was defined as synchronized, high-amplitude, low-frequency (0.4–4 Hz) EEG and highly reduced EMG activity compared with wakefulness, with no phasic bursts. REM sleep was defined as that with a pronounced theta rhythm (4–9 Hz) and a flat EMG signal (muscle atonia). Sleep deprivation After baseline sleep recording, mice were sleep-deprived for the duration indicated in each experiment (4 or 6 h), starting at light onset (ZT0). Mice were sleep-deprived by gentle handling to avoid stress responses. Analysis of Cort levels Mice were killed immediately at the end of 4 h of sleep or 4 h of sleep deprivation. Serum Cort levels were determined using a standard enzyme-linked immunosorbent assay (ELISA) for Cort (Millipore; Billerica, MA), as per the standard procedure recommended by the manufacturer. Flow cytometry Mice were killed, using CO 2 , and BM was harvested into PBS containing 2% FCS. Lineage staining was performed with fluorochrome-conjugated monoclonal antibodies (eBioscience) against Ter119 (15–5,921), Gr1 (15–5,931), Mac1 (15-0112), B220 (15-0452), CD3 (15-0031), CD4 (15-0041) and CD8 (15-0081; all in 1:200 dilution). KLS (c-Kit+, Lin−, Sca-1+) subset delineation was performed with antibodies against c-Kit (47–1,171; 1:100) and Sca-1 (17–5,981; eBioscience; 1:100). KLS proportions were evaluated in blood and BM. HSCs were determined using antibodies against CD150 (25–1,502; 1:100) and CD34 (11-0341; eBioscience; 1:25). VLA4 (103705, Biolegend; 1:100). Cells were analysed with the LSR II (BD Biosciences) or FACSAria II (BD Biosciences). HSC transplantation BM cell samples were enriched for c-kit-positive cells before staining, using anti-CD117-conjugated magnetic beads (AutoMACS, Miltenyi, Germany), according to the manufacturer’s instructions. Cells were then stained with the antibodies listed above. Cells were sorted with a FACSAria II (BD Biosciences). A total of 300 sorted putative HSCs purified from sleep controls or sleep-deprived mice and 10 6 helper BM-derived mononucleated cells (to support the survival of the mice during recovery) were transplanted into lethally irradiated (9.5 Gy γ-irradiation delivered in a split dose), 8–12-week-old congenic recipient mice via intravenous injection into the retro-orbital sinus. Peripheral blood was drawn from the tail vein of recipient mice at 8 weeks post-transplantation, and red blood cells were sedimented with 2% dextran and lysed with ammonium-chloridepotassium lysing buffer (150 mM NH 4 Cl, 1 mM KHCO 3 and 0.1 mM EDTA) for 5 min on ice. Recipient mice were killed at 16 weeks post transplantation, and whole blood was obtained by collecting the perfusate from the heart and BM was harvested by crushing bones. Donor-derived haematopoietic cells were identified with flow cytometry, using antibodies against CD45.1 (eBioscience) and host-derived haematopoietic cells were identified using anti-CD45.2 antibodies (eBioscience). There was no difference in the relative distribution of the donor cells between the blood and BM at 16 weeks. There was no difference between the two groups in mouse survival. Secondary transplantation To demonstrate the self-renewing capacity of the donor-derived long-term repopulating cells, 2.5 × 10 6 BM cells from primary recipients (who received HSCs from sleep or sleep-deprived mice) were transplanted into lethally irradiated CD45.2+ secondary recipients and donor-derived reconstitution was assessed. Of note, secondary transplant donors were not sleep-deprived before transplantation. Homing experiment FACS-purified HSCs derived from GFP-transgenic C57BL/6− CD45.1+ mice were intravenously transplanted into congenic C57BL/6-CD45.2 mice, whose bones were collected 12 h thereafter. Immunohistochemistry Bones were incubated in 4% paraformaldehyde for 24 h, washed in PBS and transferred to 400 mM EDTA for 20 days, at 4 °C, protected from light. The decalcified bones were cryoprotected overnight, at 4 °C, in 30% sucrose. Bones were sliced to a thickness of 10 μm and the number of cells expressing endogenous GFP was determined. For verification, bones were stained with anti-GFP antibody (1:1,000; Abcam; Cambridge, MA; ab13970). Binding of FITC-conjugated LDV The activation of integrin-α4β1 was determined by α 4 β 1 integrin (VLA4) coupled to fluorescein isothiocyanate (FITC; LDV-FITC) binding. Cells derived from the BM of sleep-deprived mice, and mice that were allowed to sleep were incubated for 30 min at 37 °C with 0.5 or 10 nM LDV-FITC and analysed with flow cytometry. Mx-1 and SOCS3 deletion experiment Mx-1 male 8–10-week-old mice were bred with SOCS3 floxed mice. Cre-negative mice were used as a control for potential effects of the breeding background, and the effects of intraperitoneal injections of 250 μg poly I-C (Invitrogen), which was given to induce Mx-1-mediated deletion. Poly I-C was injected three times at 24-h intervals. miR profiling Total RNA was isolated from FACS-purified HSCs, using TRIzol reagent (Invitrogen), and reverse-transcribed using MegaPlex RT primer pool A (Applied Biosystems, CA, USA). Profiling of miR expression was performed using the TaqMan Array Rodent Card A v2.0 (Applied Biosystems). The 384-well rodent array pool A plate contains four wells of U6 and snoRNA as internal controls, 335 individual highly conserved mouse miRs in each well, 45 wells of two other snoRNAs (sno-202 and sno-135) and miRs of rat and other species. Given limited amounts of RNA (<50 ng) that can be recovered from sorted HSCs, RNA was pre-amplified using TaqMan PreAmp Master Mix and PreAmp Primers (2 ×), as per the manufacturer’s protocol. Quantitative PCR cDNA was synthesized with SuperScript II Reverse Transcriptase (Invitrogen), using an anchored oligo dT primer. The samples were amplified, in duplicates, by qPCR, using TaqMan gene expression assays (Applied Biosystems) on an ABI 7900 HT system. Values were normalized to GAPDH. The following primers were used: Ghr Mm00439093; SOCS5 Mm01232423; SOCS1 Mm00782550; SOCS3 Mm01249143; hsa-miR-19a 000395; and hsa-miR-19b 000396 (all from Life Technologies). In vitro transmigration For chemotaxis assays, isolated KLS cells were suspended in migration medium comprising RPMI-1640 medium, supplemented with 0.5% BSA and then seeded in 8-μm pore transwell plates (Corning-Costar Corp). Murine SDF-1α (50, 100 or 200 ng ml −1 ; Sigma-Aldrich) or S1P (10 or 100 nM; Sigma-Aldrich) was added to the lower chamber (specific concentration is indicated for each figure). KLS cells (1 × 10 4 or 5 × 10 4 cells) were placed in the upper well and incubated at 37 °C for 4 h, and the number of cells in the lower wells was determined using flow cytometry. The migration index was calculated as the fold of increase in migration to the chemoattractant relative to baseline migration (without chemoattractant). Levels of SDF-1α and S1P were selected on the basis of previous reports [32] , [33] . Luciferase assay 293T cells (ATCC) were transfected with the 3′UTR SOCS3 luciferase construct (Origene; SC215826), miR-19 mimics and scrambled controls (based on cel-miR-67, mature sequence: 5′-UCACAACCUCCUAGAAAGAGUAGA-3′; Dharmacon), using DharmoFECT 1. Cells were analysed 48 h later, using the Luciferase Assay kit (Promega). Transfection efficiency was normalized to RFP signals. Statistical analysis Significance levels of the data were determined using Prism5 (GraphPad Software, La Jolla, CA). Experiments were analysed by two-tailed Student’s t -test or by one-way or two-way ANOVA, as indicated for each experiment. ANOVA was followed by a post hoc test. Alpha was set at 0.05. Accession codes: The miRNA microarray data have been deposited in the GEO database under accession code GSE48144 . How to cite this article: Rolls, A. et al . Sleep disruption impairs haematopoietic stem cell transplantation in mice. Nat. Commun. 6:8516 doi: 10.1038/ncomms9516 (2015).